Physical autocatalysis driven by a bond-forming thiol–ene reaction Autocatalysis has been extensively studied because it is central to the propagation of living systems. Chemical systems which self-reproduce like living cells would offer insight into principles underlying biology and its emergence from inanimate matter. Protocellular models feature a surfactant boundary, providing compartmentalization in the form of a micelle or vesicle and any model of the emergence of cellular life must account for the appearance, and evolution of, such boundaries. Here, we describe an autocatalytic system where two relatively simple components combine to form a more complex product. The reaction products aggregate into micelles that catalyse molecular self-reproduction. Study of the reaction kinetics and aggregation behaviour suggests a mechanism involving micelle-mediated physical autocatalysis and led to the rational design of a second-generation system. These reactions are driven by irreversible bond formation and provide a working model for the autocatalytic formation of protocells from the coupling of two simple molecular components. The development of chemical models of living cells is a major contemporary challenge that would find application in the field of synthetic biology [1] and bear on questions about the origins and, the very definition of, life [2] , [3] . Several designs for artificial cells have been put forward [4] , [5] , [6] , [7] , [8] . A notable and representative design proposed by Szostak, Bartel and Luisi [9] consists of ‘the union of two fundamentally different kinds of replicating systems’: a self-replicating genetic polymer encapsulated by and coupled to a self-reproducing membrane. Such a system, if realized, may serve as a useful model of the earliest life forms and could even be considered a living organism [10] , [11] , [12] , [13] . Simple chemical models of both self-replicating genetic molecules and self-reproducing membranes have been developed over the past 30 years. Given the wide interest in simple autocatalytic molecules [14] , [15] and the significant influence of the RNA world hypothesis [16] , molecules capable of template-based self-replication have been studied for many years. This field has advanced to the point that there now exist candidate substrates for the genetic material of a protocell [17] , and it has been proposed that non-enzymatic chemical replication of RNA may even be possible [18] . The self-reproduction of simple models of membranes, namely micelles and vesicles, has also been studied, most notably by Luisi and co-workers [4] . These systems represent crucial components of protocellular models and provide experimental support for ‘lipid world’ scenarios for the origins of life [19] , where catalytically active surfactant aggregates, dubbed lipozymes, act as prebiotic analogues of enzymes and under a form of selection promoted the emergence of life. Several systems are known in which surfactant aggregates catalyse chemical reactions that yield fresh surfactant molecules and thereby drive their own reproduction [14] . These reactions are autocatalytic with respect to the micelle or vesicle, a process that has been referred to as physical autocatalysis [20] , [21] , [22] , where the term autocatalysis is used in a broad sense, to refer to product-induced increase in reaction rate [4] , [14] . In contrast to the template-based replication, the type of reactions known to drive physical autocatalysis are extremely limited [14] and almost all known examples are driven by hydrolysis-mediated chemical bond cleavage [14] . To the best of our knowledge, the only examples of physical autocatalysis driven by bond-forming processes involve simple N -oxidation of an amine [23] , or imine condensation that is chemically reversible and operates under thermodynamic control [24] , [25] ( Fig. 1 ). 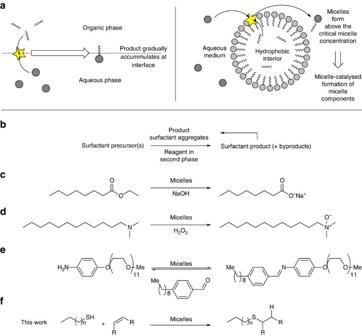Figure 1: Physical autocatalysis in micelles. (a) Schematic representation of physical autocatalysis. Species separated by a phase boundary react at the interface; the reaction is catalysed by the formation of product aggregates that allow species in each phase to mix. (b–e) Previous examples of physical autocatalysis can be divided into three classes of reaction, illustrated here with representative examples. Schemes are simplified to emphasize the reaction partners and the catalytically active product. (b) General principle of physical autocatalysis: a biphasic reaction generates surfactant products that autocatalyse the reaction; (c) Hydrolysis, typically of anhydrides, esters or imines (example from ref.35); (d) Simple oxidation (example from ref.23); (e) Reversible imine condensation under thermodynamic control (example from ref.24); (f) This work, demonstrating physical autocatalysis in an irreversible bond-forming reaction. Figure 1: Physical autocatalysis in micelles. ( a ) Schematic representation of physical autocatalysis. Species separated by a phase boundary react at the interface; the reaction is catalysed by the formation of product aggregates that allow species in each phase to mix. ( b – e ) Previous examples of physical autocatalysis can be divided into three classes of reaction, illustrated here with representative examples. Schemes are simplified to emphasize the reaction partners and the catalytically active product. ( b ) General principle of physical autocatalysis: a biphasic reaction generates surfactant products that autocatalyse the reaction; ( c ) Hydrolysis, typically of anhydrides, esters or imines (example from ref. 35 ); ( d ) Simple oxidation (example from ref. 23 ); ( e ) Reversible imine condensation under thermodynamic control (example from ref. 24 ); ( f ) This work, demonstrating physical autocatalysis in an irreversible bond-forming reaction. Full size image A simple model protocell consists of ‘core and shell’ replication. Here, either a simple self-replicating molecule or an enzymatic system is encapsulated by a self-reproducing micelle [26] , [27] or vesicle [28] , [29] . Developing a chemical protocellular model system of this kind has been a research goal for several decades; the state-of-the-art was recently and elegantly exemplified by Kurihara et al . [30] , who amplified DNA by the PCR within self-reproducing vesicles and demonstrated a coupling between the replication of nucleotides and lipids. Given the wide interest in developing protocells, we set out to explore which classes of reactions are actually capable of driving physical autocatalysis. As a starting point, we reasoned that reactions that generate molecular complexity would, at least in principle, appear to be much more relevant to the transition of simple prebiotic building blocks into living systems. Bond-forming autocatalytic systems would provide a model for the transition of simple molecules to more complex matter capable of catalytic function, as well as expand the tool kit available to protocell researchers. Synthetic reactions, where relatively simple components are brought together to make a more complex product, are arguably much more relevant to prebiotic synthesis than bond-cleaving or oxidation reactions and would allow the development of experimental tests of key claims of ‘lipid world’ scenarios. Here, by simple and complex, we are making a general observation about the molecular weight and functionality of molecules. Such reactions are a prerequisite for chemical studies of simple evolutionary processes such as selection and competition [24] analogous to the behaviour demonstrated in template-based replicators by Rebek [31] , Von Kiedrowski [32] and others [14] . Coupling processes are necessary for the combinatorial autocatalytic synthesis of a diverse population of lipids from a smaller number of precursors, whereas the use of hydrolysis reactions to generate new lipids imposes a hard limit on the number of potential lipid species in the system. To these ends, we report here a novel example of physical autocatalysis driven by irreversible bond formation. Two thiol–ene reactions are described in which the coupling of molecules of very different polarities produces an amphiphilic product, which aggregates into autocatalytically active micelles. The phase behaviour of the reaction components is studied by diffusion-ordered NMR spectroscopy (DOSY), providing some insight into the mechanism of the reaction. These systems offer a chance for novel experimental tests of key claims of the lipid world hypothesis and expand the options available for the development of protocell models. Design of self-reproducing micelles As a simple model system for complexity-generating physical autocatalytic reactions, we chose to study thiol–ene reactions [33] , the base-catalysed 1,4-conjugate addition of thiols to α,β-unsaturated carbonyls, as these are simple, selective and compatible with aqueous conditions. A candidate substrate based on a report by Matsuno et al . [34] who synthesized a library of micelle-forming phospholipids, was identified. The phospholipid was made by coupling two reactants of very different polarity, to give a stable amphiphilic product, and was deemed to be an ideal test reaction to probe physical autocatalysis ( Fig. 2 ). 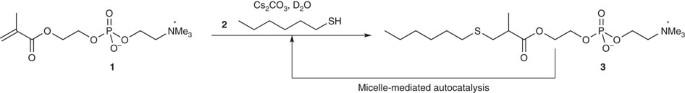Figure 2: Design of an autocatalytic model system based on a thiol–ene reaction. Substrates were previously reported by Matsunoet al.34The biphasic reaction of1and2produces3. As3forms micelles above 25 mM, it was expected to catalyse the reaction, and hence the reaction was predicted to be autocatalytic. Figure 2: Design of an autocatalytic model system based on a thiol–ene reaction. Substrates were previously reported by Matsuno et al . [34] The biphasic reaction of 1 and 2 produces 3 . As 3 forms micelles above 25 mM, it was expected to catalyse the reaction, and hence the reaction was predicted to be autocatalytic. Full size image Our initial approach to this system was intended to be as straightforward as possible. As such, we imitated the reaction conditions used by Bachmann et al . [35] in their classic paper establishing physical autocatalysis in micelles: two clearly separated phases, stirred gently and monitored by removal of aliquots. Other authors studying physical autocatalysis have opted to rapidly mix the two phases to reduce the reaction time [36] ; our choice was based on several considerations, particularly the desire to sample the aqueous phase directly and thereby minimize the amount of thiol present in the NMR tube to improve spectral quality. After preliminary experimentation, we found that when a solution of 2-methacryloyloxyethyl phosphorylcholine 1 in D 2 O at high pH is gently stirred with hexanethiol 2 , autocatalytic behaviour is observed ( Fig. 3 ). The high pD of the reaction leads to rapid but self-limiting hydrolysis of 1 to methacrylate within the first minutes of the reaction (see Supplementary Figs 1–3 ). After about 20% hydrolysis, the Michael acceptor is stable to further degradation and autocatalytic 1,4-addition of 2 is then observed. 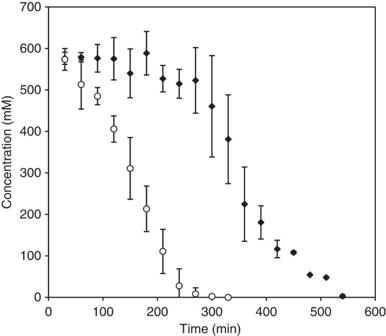Figure 3: Evidence of autocatalysis in the reaction of1and2. The reaction is monitored by disappearance of1by1H NMR spectroscopy. Data points are the mean of three experiments and error bars show the s.d. ♦ Control reaction: when1and2are stirred gently, a lag period followed by a faster reaction period is observed.○Seeded reaction: when the reaction is seeded with3att=0, the lag period is eliminated and the reaction proceeds in a more linear fashion. Representative stacked spectra are shown inSupplementary Figs 6 and 7. Figure 3: Evidence of autocatalysis in the reaction of 1 and 2 . The reaction is monitored by disappearance of 1 by 1 H NMR spectroscopy. Data points are the mean of three experiments and error bars show the s.d. ♦ Control reaction: when 1 and 2 are stirred gently, a lag period followed by a faster reaction period is observed. ○ Seeded reaction: when the reaction is seeded with 3 at t =0, the lag period is eliminated and the reaction proceeds in a more linear fashion. Representative stacked spectra are shown in Supplementary Figs 6 and 7 . Full size image Autocatalysis in the conjugate addition is suggested by two observations characteristic of autocatalytic processes [14] . The first of these is an increase in the rate of the reaction following a lag period ( Fig. 3 , black circles). The second observation supporting the autocatalytic behaviour is that the reaction rate increases when 20 mol% (130 mM, critical micelle concentration (cmc)=25 mM (ref. 34 )) of the product is added at the start of the reaction ( Fig. 3 , white circles). This behaviour is reproducible (see Supplementary Fig. 4 ) and, consistent with the detailed kinetic studies of related reactions [36] , sensitive to various physical factors including the size and orientation of the stirrer bar, the rate of stirring, and the shape of the reaction flask (see Supplementary Fig. 5 ). The mechanism by which physical autocatalysis proceeds has been debated. Early work on self-reproducing micelles assumed that these reactions proceed through micellar catalysis, but this was disputed by Buhse et al . [36] , [37] The latter developed kinetic models and concluded that physical autocatalysis can be thought of as a form of phase transfer catalysis. Essentially, the difference between the two models is in the location of the key reaction: Luisi et al . assumed that the reaction occurred at the micelle, while Buhse et al . provide evidence that the surfactant precursor is released from micelles into the aqueous phase to react in bulk solution. NMR studies We opted to use DOSY to study this reaction. This technique has been used to study the formation of micelles and uptake of solutes into micelles for several decades, and provides insight into aggregation phenomena by measuring the self-diffusion coefficient of molecules, which is strongly correlated with the average size and shape of a species or an aggregate [38] , [39] . Nguyen et al . [24] used DOSY in their study of self-reproducing micelles but as their starting materials and product are in equilibrium, the concentrations of components cannot be adjusted independently. As the thiol–ene reaction described here is irreversible, we were able to take our DOSY study further and show how aggregation of individual reaction components varies with concentration. Our first step was to confirm the cmc of 3 by DOSY. This was reported by Matsuno et al . to be 25 mM as determined by surface tension measurements; by DOSY, we measure a cmc of 26.5 mM, in close agreement (see Supplementary Fig. 8 ). Following this we repeated the measurement in the presence of 2 (100 mM) to see if mixed micelles of the thiol and lipid have a significantly lower cmc. Under these conditions we measured a cmc of 23.4 mM, consistent with favourable formation of mixed micelles of 3 and 2 (ref. 36 ). It is clear from the diffusion coefficient ( D ) values ( Table 1 ) obtained for 2 in the presence and absence of 3 that, in the presence of micelles of 3 , 2 is significantly solubilized ( Fig. 4 ). Using a method reported by Stilbs [40] , which uses tetramethylsilane (TMS) as a reporter molecule for micellar diffusion coefficient, we calculated the degree of solubilization of 2 into micelles of 3 ([ 3 ]=100 mM) as >99%. On this basis, we would tentatively like to conclude that our system largely operates by the micellar catalysis mechanism proposed by Luisi, rather than a phase transfer mechanism as described by Buhse et al . [36] Table 1 Uptake of 2 into micelles of 3. 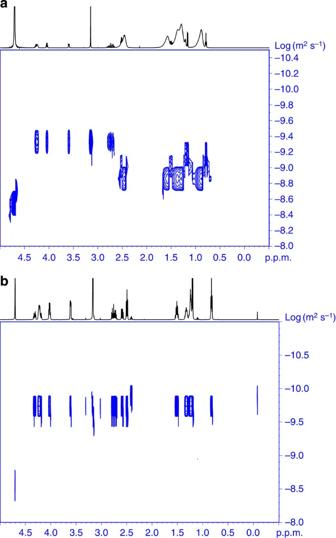Figure 4: DOSY NMR showing uptake of2into micelles of3. (a) 2D DOSY spectrum shows the difference inDfor2and3. Peaks between 2.5–0.5 p.p.m. correspond to protons of2and the alkyl chain of3, with an isolated triplet at 2.42 p.p.m. providingDfor2. Experiment performed on a mixture of3(1 mM) and2(saturated); (b) 2D DOSY spectrum shows the coincidence of diffusion coefficients for2,3and TMS. Experiment performed on a mixture of3(100 mM),2(saturated) and TMS (saturated). See alsoSupplementary Fig. 9. Full size table Figure 4: DOSY NMR showing uptake of 2 into micelles of 3 . ( a ) 2D DOSY spectrum shows the difference in D for 2 and 3 . Peaks between 2.5–0.5 p.p.m. correspond to protons of 2 and the alkyl chain of 3 , with an isolated triplet at 2.42 p.p.m. providing D for 2 . Experiment performed on a mixture of 3 (1 mM) and 2 (saturated); ( b ) 2D DOSY spectrum shows the coincidence of diffusion coefficients for 2 , 3 and TMS. Experiment performed on a mixture of 3 (100 mM), 2 (saturated) and TMS (saturated). See also Supplementary Fig. 9 . Full size image Unfortunately, the applicability of these results to our reaction conditions is not clear. The high pH of the reaction means that significant quantities of thiolate ion are present. These would be expected to be significantly more soluble in water than the thiol and hence the degree of solubilization into the micelle may be lower. Further, the higher ionic strength due to the presence of Cs 2 CO 3 may well affect the aggregation properties of 3 . We opted not to repeat the DOSY study at high pD as any hydrolysis of 3 would affect the obtained diffusion coefficients, and the higher ionic strength of the solution gave poor spectral resolution in preliminary measurements, leading to overlap of peaks of 2 and 3 . Design of a second-generation system With these issues in mind, we decided to rationally design a second-generation system. We envisaged that a more reactive alkene would give higher levels of reactivity. This may allow reaction under milder conditions and/or at lower concentrations, and possibly allow the use of longer thiols, which we found were quite unreactive with the above system. Further, a reaction carried out at neutral pH would allow our DOSY study to be directly applicable to the reaction conditions. Lipid precursor 4 contains a maleimide, widely used in bioconjugation reactions [41] ( Fig. 5 ). 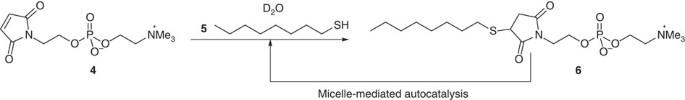Figure 5: Second-generation autocatalytic thiol–ene reaction. The biphasic reaction of4and5produces6. As6forms micelles above 5 mM, it was expected to catalyse the reaction, and hence the reaction was predicted to be autocatalytic. The use of a maleimide as the Michael acceptor allows the reaction to proceed under conditions more relevant to model protocells. Figure 5: Second-generation autocatalytic thiol–ene reaction. The biphasic reaction of 4 and 5 produces 6 . As 6 forms micelles above 5 mM, it was expected to catalyse the reaction, and hence the reaction was predicted to be autocatalytic. The use of a maleimide as the Michael acceptor allows the reaction to proceed under conditions more relevant to model protocells. Full size image When a solution of maleimide 4 in D 2 O (21 mM Tris buffer, pD 7.85) is gently stirred with octanethiol 5 , autocatalytic behaviour is again observed ( Fig. 6 ). The reaction was found to be sensitive to pD; below 7, the reaction hardly proceeds, and above pD 7.9 some (~5%) hydrolysis of the maleimide is observed. As before, autocatalysis is suggested by an increase in the rate of reaction following a lag period, and the elimination of this lag period by the addition of lipid 6 at the start of the reaction. 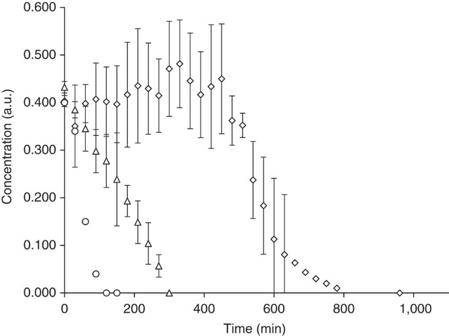Figure 6: Evidence of autocatalysis in the reaction of4and5. The reaction is monitored by disappearance of4by1H NMR spectroscopy. Data points are the mean of three experiments and error bars show the s.d.⋄Control reaction: when4and5are stirred gently, a lag period followed by a faster reaction period is observed. Δ Seeded reaction: when the reaction is seeded with 20 mol%6att=0, the lag period is eliminated and the reaction proceeds linearly.○Seeded reaction (single experiment): addition of 70 mol% of6att=0 further increases the rate of reaction. Representative stacked spectra are shown inSupplementary Figs 10 and 11. Figure 6: Evidence of autocatalysis in the reaction of 4 and 5 . The reaction is monitored by disappearance of 4 by 1 H NMR spectroscopy. Data points are the mean of three experiments and error bars show the s.d. ⋄ Control reaction: when 4 and 5 are stirred gently, a lag period followed by a faster reaction period is observed. Δ Seeded reaction: when the reaction is seeded with 20 mol% 6 at t =0, the lag period is eliminated and the reaction proceeds linearly. ○ Seeded reaction (single experiment): addition of 70 mol% of 6 at t =0 further increases the rate of reaction. Representative stacked spectra are shown in Supplementary Figs 10 and 11 . Full size image That the lag period is longer than in the above system is readily explained by the lower solubility of octanethiol in neutral D 2 O than hexanethiol in alkaline D 2 O. However, on the formation of quantities of 6 in excess of its cmc, the reaction proceeds at a similar rate to the first-generation system, reflecting the higher reactivity of the maleimide. The large s.d. of peaks in the linear reaction phase are an artefact of the fact that each reaction reaches this phase at a slightly different time; the raw data are plotted in the SI. NMR studies of the second-generation system The cmc of 6 was measured as 4.8 mM by DOSY NMR (see Supplementary Fig. 8 ). As before, the study of the maleimide-based system by DOSY NMR ( Fig. 7 ) clearly shows that 5 is entirely bound within 6 when 6 is present in a large excess of its cmc ( Table 2 ). In this case, we studied the aggregation behaviour at a greater range of concentrations, and confirmed that the maleimide starting material 4 neither aggregates nor is taken into the micelles of 6 ( Table 2 , rows I–K). 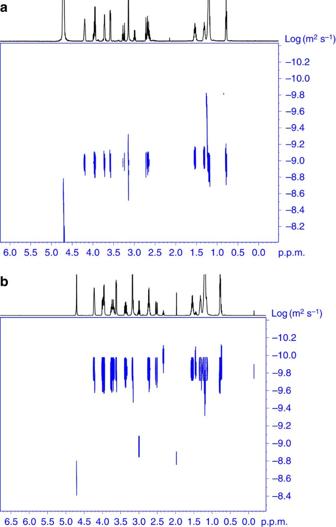Figure 7: DOSY NMR showing uptake of5into micelles of6. (a) 2D DOSY spectrum shows rapid diffusion of6. No5was directly observed in this experiment despite the solution being saturated before measurement. Experiment performed on a mixture of6(2 mM) and5(saturated; corresponding toTable 2row D); (b) 2D DOSY spectrum shows the coincidence of diffusion coefficients for5,6and TMS. Experiment performed on a mixture of6(50 mM),2(saturated) and TMS (saturated; corresponding toTable 2row H). See alsoSupplementary Fig. 12. Figure 7: DOSY NMR showing uptake of 5 into micelles of 6 . ( a ) 2D DOSY spectrum shows rapid diffusion of 6 . No 5 was directly observed in this experiment despite the solution being saturated before measurement. Experiment performed on a mixture of 6 (2 mM) and 5 (saturated; corresponding to Table 2 row D); ( b ) 2D DOSY spectrum shows the coincidence of diffusion coefficients for 5 , 6 and TMS. Experiment performed on a mixture of 6 (50 mM), 2 (saturated) and TMS (saturated; corresponding to Table 2 row H). See also Supplementary Fig. 12 . Full size image Table 2 Uptake of 5 into micelles of 6. Full size table In the presence of sub-cmc concentrations of 6 , thiol 5 is not readily detectible by 1 H NMR ( Table 2 , row D); trace quantities were seen in the two-dimensional (2D) DOSY spectrum but diffusion coefficients could not be obtained from these data. This decrease in solubility in the presence of 6 compared to a solution of pure 5 may be due to a salting-out effect. In the presence of 50 mM 6 (~10 times the cmc; Table 2 , row H) 5 is completely bound to slow-diffusing aggregates. Unexpectedly, under these conditions, 5 was found to have a lower D than that of TMS. The Stilbs method [40] assumes that TMS is fully bound to micelles and hence takes its D as an approximation of the ideal diffusion of micelles, as the observed diffusion coefficient of lipids is an average of the free and aggregated lipid. In the case of lipid 6 , thiol 5 was found to have an even smaller diffusion coefficient than TMS. These experiments strongly suggest that 5 is completely bound to micelles of 6 , that is, all 5 is either in a bulk thiol layer or contained within micelles. Despite this limitation, we studied the uptake of thiol at intermediate concentrations at and above the cmc ( Table 2 , rows E–G). As can be seen from Table 2 , in the cmc region (5–10 mM), there is an appreciable concentration of free lipid compared with experiments at higher lipid concentrations, but the thiol is strongly bound even at a small excess of the cmc. We therefore conclude that this reaction is unlikely to proceed via a phase transfer mechanism as described by Buhse et al . [36] Thiol 5 is negligibly soluble in aqueous solution and as the concentration of lipid 6 increases beyond the cmc, the diffusion coefficient of 5 continues to decrease as it binds tightly to growing micelles of 6 . This suggests that the reaction occurs in association with the micelles, matching closely the mechanism proposed by Luisi and Varela [42] . The first studies of self-reproducing micelles reported by Luisi were an explicit attempt to develop a minimal autopoietic system. Autopoiesis is a definition of the minimal criteria for life originally proposed by Maturana and Varela [43] describing a system, defined by a boundary, that encapsulates all of the processes needed to produce all of the components of the system [12] . This system is also a minimal model of autopoiesis, consisting of one component (lipid 6 ) that forms a boundary encapsulating the reaction that generates 6 . Whether or not minimal autopoietic systems actually meet the minimal criteria for life is disputed even by proponents of autopoiesis [2] , [12] . ‘Lipid world’ scenarios of the origins of life have been assessed extensively in silico [44] but experimental support remains limited. The use of coupling reactions to generate new lipids irreversibly provides the conceptual basis for experimental tests of ‘lipid world’ models by allowing the combinatorial synthesis of heterogeneous populations of lipid assemblies. Diverse lipid populations of this kind are prerequisites for models of competition and selection amongst physical autocatalysts relevant to the origins of life. As such, the novel reactions reported here may allow experimental testing of proposed prebiotic chemistry. In summary, we have described two examples of physical autocatalysis driven by thiol–ene chemistry. These are the first examples of physical autocatalysis driven by irreversible bond formation and as such represent both a novel technology for the study of model protocells and a model for the autocatalytic generation of functional complex molecules under prebiotic conditions. We anticipate autocatalytic coupling reactions will aid new experimental models of prebiotic chemistry and in the development of model protocells. General experimental All chemicals and solvents were purchased from Sigma Aldrich or Apollo Scientific and used without further purification. All NMR spectra were recorded at room temperature. NMR spectra were recorded using Bruker DPX-200 (200 MHz), DPX-250 (250 MHz), DRX-500 (500 MHz) or AVC-500 (500 MHz) spectrometers. 13 C and 31 P NMR spectra were recorded using Bruker AVC-500 (500/125 MHz) and DRX-500 (500/200 Mhz) spectrometers, respectively. Chemical shifts are reported in p.p.m. from the residual solvent peak. Chemical shifts ( δ ) are given in p.p.m. and coupling constants ( J ) are quoted in hertz (Hz). Resonances are described as s (singlet), d (doublet), t (triplet), q (quartet) and m (multiplet). High-resolution mass spectra were recorded using a Bruker MicroTOF spectrometer by the internal service at the University of Oxford. 1 H NMR spectra of key reagents can be seen in Supplementary Figs 14–17 pD measurements of samples in D 2 O were made using a Jenway 3510 pH meter calibrated using standard reference samples in H 2 O. pD values were estimated from the observed pH* values according to Krżel and Bal [45] . DOSY NMR measurements were performed using a Bruker AVII-500 equipped with a TFI probehead at 298 K using the 2D sequence for diffusion measurement using double stimulated echo for convection compensation and longitudinal eddy current delay, using bipolar gradient pulses for diffusion, and using three spoil gradients (Bruker terminology: dstebpgp35) pulse sequence [46] , [47] . The samples were thoroughly mixed using a Vortex Genie 2 mixer (Scientific Industries), and were then clarified using a hand centrifuge (Hettich, model 1011) and then measured. Samples containing saturated thiol consequently had a small layer of neat thiol above the D 2 O layer; sufficient D 2 O was used to ensure that the thiol layer was not detectible by the NMR probe. Experiments were performed in two stages: initially 1D-edited DOSY experiments were used to optimize the diffusion period Δ for each of 3 (Δ=150 ms) and 6 (Δ=170 ms). The 2D dstebpgp35 sequence was then used, based on the optimized Δ from the previous procedure and with δ=4 ms, with gradient amplitude ranging from 2 to 85% with 16 points in between. Data were analysed using the T1T2 module in TOPSPIN 3.2 and plots were generated using the eddosy module. Synthesis of compound 3 Compound 3 was synthesized according to Matsuno et al . [34] From 1 (2.50 g, 8.47 mmol) and 2 (1.30 ml, 9.15 mmol, 1.08 eq) in EtOH (10 ml) was obtained pure 3 (2.45 g, 5.92 mmol, 70%). 1 H NMR (500 MHz, CD 3 OD) δ 4.20–4.36 (m, 4 H), 4.08 (dt, J =7.0, 4.9 Hz, 2 H), 3.60–3.69 (m, 2 H), 3.24 (s, 9 H), 2.80 (dd, J =13.7, 7.4 Hz, 1 H), 2.71 (ddq, J =13.7, 12.8, 7.0, 7.0, 7.0 Hz, 1 H), 2.60 (dd, J =12.9, 6.3 Hz, 1 H), 2.53 (t, J =7.3 Hz, 2 H), 1.56 (quin, J =7.4 Hz, 2 H), 1.26–1.45 (m, 6 H), 1.24 (d, J =6.9 Hz, 3 H), 0.91 (t, J =7.0 Hz, 3 H); 13 C NMR (125 MHz, CD 3 OD) δ 176.86, 67.49 (dt, J =7.4, 3.1 Hz), 65.26 (d, J =7.9 Hz), 64.71 (d, J =5.5 Hz), 60.47 (d, J =5.0 Hz), 54.76 (t, J =3.8 Hz, 3 C), 41.63, 36.31, 33.44, 32.62, 30.74, 29.57, 23.68, 17.25, 14.45; 31 P NMR (200 MHz, CD 3 OD) δ p.p.m. 0.81; high-resolution mass spectrometry electrospray ionization (HRMS (ESI)) m/z calcd for C 17 H 36 NNaO 6 PS [M+Na] + : 436.1893, found: 436.1892. Synthesis of compound 4 N -Hydroxyethyl maleimide was synthesized according to Heath et al . [48] From maleic anhydride (40.0 g, 407.9 mmol) was obtained pure N -hydroxyethyl maleimide (8.34 g, 59.1 mmol, 14.5% yield over three steps). 1 H NMR (400 MHz, (CD 3 ) 2 SO) δ 7.01 (s, 2 H), 4.79 (m, 1 H), 3.46 (m, 4 H); 13 C NMR (101 MHz, (CD 3 ) 2 SO) δ 171.1, 134.5, 75.0, 57.9; MS (ESI) m/z 164.1 [M+Na] + . A solution of N -hydroxyethyl maleimide (4.30 g, 30.5 mmol) and triethylamine (6.4 ml, 45.7 mmol, 1.5 eq) in dry tetrahydrofuran (200 ml) was cooled to 0 °C and 2-chloro-1,3,2-dioxaphospholane 2-oxide (3.2 ml, 33.5 mmol, 1.1 eq) was added dropwise. The reaction was allowed to warm to room temperature and to react until complete consumption of starting material (TLC control, EtOAc). The reaction mixture was filtered through SiO 2 (eluting with EtOAc) and concentrated to a solid white residue. The crude solid was added under Ar to a 100 ml pressure tube containing a stirrer bar and dry MeCN (80 ml) was added. The tube was cooled to −20 °C and freshly distilled NMe 3 (2 ml, excess), stored at −78 °C, was added. The tube was quickly sealed and then heated to 80 °C overnight. On cooling to room temperature, the MeCN was decanted and a red precipitate, crude 4 , was purified by two rounds of SiO 2 column chromatography in EtOAc/MeOH/H 2 O/AcOH (8:8:3:1) and MeCN/H 2 O (7:3), respectively to give pure 4 (2.8 g, 30%). 1 H NMR (700 MHz, CD 3 OD) δ 6.83 (s, 2 H), 4.24 (m, 2 H), 4.01 (dt, J =6.2, 5.6 Hz, 2 H), 3.74 (t, J =5.7 Hz, 2 H), 3.63 (m, 2 H), 3.22 (s, 9 H); 13 C NMR (176 MHz, CD 3 OD) δ 172.6, 135.3 (m), 67.6 (m), 63.6 (d, J =5.1 Hz), 60.6 (d, J =5.1 Hz), 54.8 (m), 39.5 (d, J =7.9 Hz); 31 P NMR (202 MHz, CD 3 OD) δ 0.94; HRMS (ESI) m/z calcd for C 11 H 19 N 2 NaO 6 P [M+Na] + : 329.0873, found: 329.0868. Synthesis of compound 6 Compund 4 (500 mg, 1.6 mmol) and octanethiol 5 (0.32 ml, 1.8 mmol, 1.1 eq) were dissolved in EtOH (10 ml) and diisopropylamine (catalytic) was added. The reaction was stirred at room temperature until complete consumption of 4 (TLC control, MeCN/H 2 O 7:3). The solvent was evaporated and the residue washed with hexane (3 × 10 ml) and then freeze-dried to give pure 6 (701 mg, 95.9%). 1 H NMR (700 MHz, D 2 O) δ 4.25 (br m, 2 H), 4.03 (dd, J =9.0, 4.1 Hz, 1 H), 4.00 (q, J =5.7 Hz, 2 H), 3.77 (m, 2 H), 3.63 (m, 2 H), 3.31 (dd, J =18.9, 8.9 Hz, 1 H), 3.19 (s, 9 H) 2.72 (m, 3 H), 1.59 (dq, J =13.8, 7.0 Hz, 2 H), 1.36 (m, 2 H), 1.18–1.32 (m, 8 H), 0.83 (t, J =6.88 Hz, 3 H); 13 C NMR (176 MHz, D 2 O) δ 179.7, 178.3, 66.0 (m), 61.9 (d, J =5.1 Hz), 59.5 (d, J =5.1 Hz), 54.0 (t, J =4.1 Hz), 40.1, 39.6 (d, J =7.6 Hz, 9 C), 36.2, 31.1, 30.6, 28.4, 28.3, 28.2, 27.8, 22.0, 13.4; 31 P NMR (202 MHz, D 2 O) δ 0.88; HRMS (ESI) m/z calcd for C 19 H 37 N 2 NaO 6 PS [M+Na] + : 475.2002, found: 475.2011. Autocatalytic reaction of 1 and 2 A stock solution of 1 (680 mM), Cs 2 CO 3 (200 mM), MeCN (100 mM, 0.15 eq) and optionally 3 (134 mM, 0.2 eq, >5 × cmc) in D 2 O was prepared and allowed to stand for 5 min. It was then divided into 2 ml portions in cylindrical 20 × 70 mm vials with octagonal 15 × 5 mm magnetic stirrer bars. 1-Hexanethiol 3 (1.9 ml, 13.6 mmol, 10 eq) was added to each vial by ejection from a syringe down the side of the vial so as not to disturb the aqueous layer. The biphasic mixture was stirred at 150 r.p.m. as determined by the digital readout of an IKA Basic stirrer/hotplate. Aliquots (0.05 ml) were withdrawn from the aqueous layer and quenched by dilution with 0.6 ml D 2 O, and analysed by 1 H NMR spectroscopy on a 250 or 200 MHz machine. Peaks were integrated relative to MeCN (2.06 p.p.m.). Autocatalytic reaction of 4 and 5 A stock solution of 4 (100 mM), MeCN (100 mM) and optionally 6 (20 or 70 mM) in buffered (21 mM Tris, pD 7.85) D 2 O was prepared. It was then divided into 3 ml portions in cylindrical 20 × 70 mm vials with octagonal 15 × 5 mm magnetic stirrer bars. 1-Octanethiol 5 (0.53 ml, 10 eq) was added to each vial by ejection from a syringe down the side of the vial so as not to disturb the aqueous layer. The biphasic mixture was stirred at 150 r.p.m. as determined by the digital readout of an IKA Basic stirrer/hotplate. Aliquots (0.05 ml) were withdrawn from the aqueous layer and quenched by dilution with 0.6 ml D 2 O and analysed by 1 H NMR spectroscopy on a 400 MHz machine. Peaks were integrated relative to MeCN (2.06 p.p.m. ). How to cite this article: Bissette, A. J. et al . Physical autocatalysis driven by a bond-forming thiol–ene reaction. Nat. Commun. 5:4607 doi: 10.1038/ncomms5607 (2014).